Persistent spin excitations in doped antiferromagnets revealed by resonant inelastic light scattering How coherent quasiparticles emerge by doping quantum antiferromagnets is a key question in correlated electron systems, whose resolution is needed to elucidate the phase diagram of copper oxides. Recent resonant inelastic X-ray scattering (RIXS) experiments in hole-doped cuprates have purported to measure high-energy collective spin excitations that persist well into the overdoped regime and bear a striking resemblance to those found in the parent compound, challenging the perception that spin excitations should weaken with doping and have a diminishing effect on superconductivity. Here we show that RIXS at the Cu L 3 -edge indeed provides access to the spin dynamical structure factor once one considers the full influence of light polarization. Further we demonstrate that high-energy spin excitations do not correlate with the doping dependence of T c , while low-energy excitations depend sensitively on doping and show ferromagnetic correlations. This suggests that high-energy spin excitations are marginal to pairing in cuprate superconductors. Initial Cu L 3 -edge resonant inelastic X-ray scattering (RIXS) measurements on undoped and weakly underdoped cuprates [1] , [2] complemented earlier neutron and Raman scattering experiments, seeming to favour a spin-fluctuation scenario as a viable explanation of superconductivity [3] . However, more recent RIXS measurements on overdoped cuprates [3] , [4] , [5] , [6] have shown persistent high-energy spin excitations to very high doping levels where superconductivity disappears. In contrast neutron and Raman measurements display an absence of robust spin excitations in the overdoped regime [7] , [8] ; this conflict undermines an understanding of unconventional superconductivity in the cuprates, making an investigation of how spin excitations manifest in the RIXS cross-section a crucial component to its resolution. In this letter, we reconcile these seemingly incompatible experimental results by computing Cu L 3 -edge RIXS spectra using exact diagonalization (ED), capable of reproducing major experimental features. We demonstrate with light polarization analysis that the RIXS cross-section in a crossed-polarization geometry can be interpreted simply in terms of the spin dynamical structure factor S ( q , ω), which enables a comparison between different scattering experiments. Utilizing determinant quantum Monte Carlo (DQMC), we study in detail the momentum and doping dependence of S ( q , ω), finding strong changes near both (π, π) and (0, 0) with relatively insensitive antiferromagnetic zone boundary (AFZB) paramagnons upon hole doping. Moreover, with electron doping these same AFZB paramagnons harden significantly, which has recently been confirmed experimentally. Underlying this observed behaviour is a framework of local spin exchange, which remains robust even with significant doping away from the parent antiferromagnet. In contrast, our calculations show a sensitive evolution of low-energy paramagnons near (0, 0) and (π, π), which give evidence for the predominance of ferromagnetic correlations. These results highlight the importance of spectral weight and dispersion at low energies in establishing a relevant energy scale and strength of spin fluctuations for pairing rather than higher-energy AFZB paramagnons. The relationship between RIXS and S ( q , ω ) RIXS is a resonant technique and its sensitivity to magnetic excitations arises as a result of core-level spin-orbit interactions in the intermediate state (see Fig. 1a ). Although in Mott insulators it has been shown that the RIXS cross-section can be approximated by S ( q , ω) when the charge excitations are gapped, it is not clear whether the same approximation carries over to doped systems where the ground state is no longer that of a Mott insulator with commensurate filling [9] , [10] . 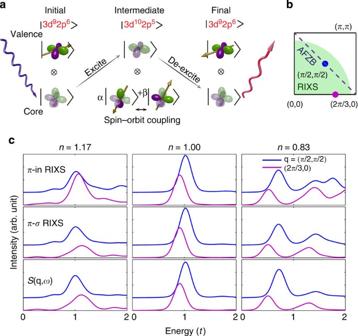Figure 1: Similarities between RIXS and the spin dynamical structure factorS(q,ω). (a) Schematic diagram of a spin-flip excitation produced during the RIXS process at the CuL3-edge. The highlighted (darkened) orbitals represent holes. A spin-flip excitation is created when an electron with up spin is photoexcited from a Cu 2pcore-level into the partially filledorbital. Subsequent de-excitation through the decay of an electron with down spin into the core produces a RIXS cross-section with a single spin-flip excitation. Such a single spin-flip channel can only be enabled when the outgoing photon polarization is (or has non-zero component) perpendicular to the incoming photon polarization. (b) A schematic picture of the area of the Brillouin zone accessible to RIXS at the CuL-edge, as well as a line denoting the antiferromagnetic zone boundary (AFZB). The RIXS cross-section and the spin dynamical structure factorS(q, ω) have been evaluated in momentum space at the points marked by dots in the Brillouin zone (see also panel (c) below). (c) The RIXS cross-section for select points in momentum space at the CuL3-edge (top and middle panels) compared againstS(q, ω) (bottom panels). Each has been calculated using exact diagonalization for the Hubbard model on a finite-size cluster for three different electron concentrationsn. The top panels show RIXS spectra calculated for an in-coming polarization π and a sum over the outgoing polarizations. The middle panels show the results with out-going polarization discrimination, here chosen in the cross-polarized geometry to emphasize the spin excitations. The results were obtained for the Hubbard model parametersU=8t,t′=−0.3twitht=0.4 eV, a Lorentzian broadening with half width at half maximum (HWHM)=0.025tand a Gaussian broadening with HWHM=0.118ton the energy transfer (see Methods). Figure 1: Similarities between RIXS and the spin dynamical structure factor S ( q , ω ). ( a ) Schematic diagram of a spin-flip excitation produced during the RIXS process at the Cu L 3 -edge. The highlighted (darkened) orbitals represent holes. A spin-flip excitation is created when an electron with up spin is photoexcited from a Cu 2 p core-level into the partially filled orbital. Subsequent de-excitation through the decay of an electron with down spin into the core produces a RIXS cross-section with a single spin-flip excitation. Such a single spin-flip channel can only be enabled when the outgoing photon polarization is (or has non-zero component) perpendicular to the incoming photon polarization. ( b ) A schematic picture of the area of the Brillouin zone accessible to RIXS at the Cu L -edge, as well as a line denoting the antiferromagnetic zone boundary (AFZB). The RIXS cross-section and the spin dynamical structure factor S ( q , ω) have been evaluated in momentum space at the points marked by dots in the Brillouin zone (see also panel ( c ) below). ( c ) The RIXS cross-section for select points in momentum space at the Cu L 3 -edge (top and middle panels) compared against S ( q , ω) (bottom panels). Each has been calculated using exact diagonalization for the Hubbard model on a finite-size cluster for three different electron concentrations n . The top panels show RIXS spectra calculated for an in-coming polarization π and a sum over the outgoing polarizations. The middle panels show the results with out-going polarization discrimination, here chosen in the cross-polarized geometry to emphasize the spin excitations. The results were obtained for the Hubbard model parameters U =8 t , t ′=−0.3 t with t =0.4 eV, a Lorentzian broadening with half width at half maximum (HWHM)=0.025 t and a Gaussian broadening with HWHM=0.118 t on the energy transfer (see Methods). Full size image To answer this question, we numerically evaluate the RIXS cross-section as a function of momentum ( Fig. 1c ) directly from the Kramers-Heisenberg formula [11] , [12] using small cluster ED of an effective single-band Hubbard Hamiltonian (including both nearest t and next-nearest neighbour hopping t ′ and on-site Coulomb repulsion U ) at various electron concentrations n ; details are given in the Methods section. Figure 1c displays the RIXS spectra calculated for the experimental geometry discussed in ref. 3 . The RIXS spectra, even without outgoing polarization discrimination, agree well with S ( q , ω) for different electron concentrations at the chosen momentum space points accessible on the same finite size clusters for each calculation. This is particularly true at half-filling where the charge gap ensures that only spin excitations can be visible in the given energy range. The main differences occur in the doped systems at higher energy (close to 2 t ), which are of less interest for our spin analysis. The important result shown in Fig. 1c concerns the suppression of these higher energy peaks in the cross-polarized geometry (see Fig. 1c π−σ RIXS) which leads to a significant improvement in the comparison between the RIXS cross-section and S ( q , ω). This indicates that Cu L 3 -edge RIXS with crossed polarizations (a four-particle correlator) provides access to the spin excitation spectrum encoded in S ( q , ω) (a two-particle correlator) for doped as well as undoped cuprates. (To further confirm this agreement between RIXS and S ( q , ω) for more momentum points, we manually adjusted the Cu L -edge energy to be 1.8*930 eV=1674, eV so that momentum points up to (π, π) can be reached. For more details see Supplementary Note 1 .) The momentum and doping dependence of S ( q , ω ) Having established a relationship between RIXS and S ( q , ω), we focus now on the momentum and doping dependence of S ( q , ω) for the single-band Hubbard model. Here we employ the numerically exact DQMC method (see Methods) with maximum entropy analytic continuation on larger lattices with fine control of the electron concentration through the chemical potential. As shown in Fig. 2 the DQMC calculations qualitatively reproduce both the momentum and doping evolution of the RIXS measurements found in refs 1 , 2 , 3 , 4 , 5 , 6 . A comparison between the intensity and dispersion of low-energy magnetic excitations near (0, 0) and (π, π) shows a transition from antiferromagnetic to ferromagnetic spin correlations with increasing doping. [In an antiferromagnetic system, the dynamical spin structure factors show gapless excitations at both (0, 0) and (π, π), with strong intensity around (π, π). In a ferromagnetic system, the dynamical spin structure factors show strong intensity with gapless excitations at (0, 0) and much weaker intensity with gapped excitations when approaching (π, π)]. However, the spectra of higher-energy AFZB paramagnons show relatively little change with hole doping other than a general decrease of intensity, suggesting that spin excitations do not soften even in the heavily overdoped regime. For electron doping, AFZB paramagnons surprisingly harden by 50% at 15% doping that has been observed recently in the prototypical electron-doped cuprate Nd 2− x Ce x CuO 4 (ref. 13 ). For additional analysis and discussion, see Supplementary Discussion . Theory to understand AFZB paramagnons The behaviour of these AFZB paramagnons stands in stark contrast to naive expectations of spin softening with either hole or electron doping: (i) long-range AF order collapses quickly upon doping with a small (intermediate) concentration of holes (electrons), and one would expect spin excitations to soften accordingly [14] , [15] ; (ii) short-range AF correlations are further weakened due to a dilution of AF bonds (see Fig. 3a ) in the locally static spin picture. Indeed, the nearest neighbour spin-spin correlations from the DQMC calculations with electron doping decrease in a manner surprisingly well described by a locally static spin picture where the doped electrons are immobile, as shown in Fig. 3b . 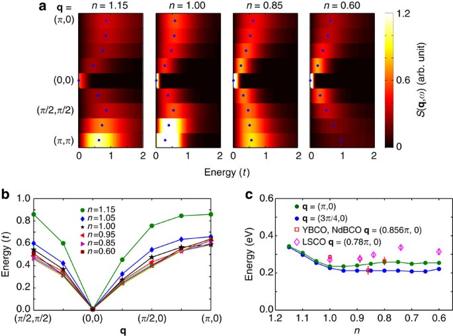Figure 2: The spin dynamical structure factorS(q,ω) calculated using DQMC for the Hubbard model. (a) False colour plots of the spectra along high symmetry directions in the Brillouin zone for different electron concentrationsn. The calculations are done with the same Hubbard model parameters as inFig. 1. (b) Dispersion relations of the spin response peak inS(q, ω) along these high symmetry directions for differentn. (c) Comparison of the calculated and observed energies of the spectral peaks at selected momenta as a function ofn(t=400 meV has been used for the comparison). YBa2Cu3O6+x, YBa2Cu4O8and Nd1.2Ba1.8Cu3O6+xRIXS experimental data are taken from ref.3; La2−xSrxCuO4RIXS experimental data are taken from ref.6. Error bars on the experimental data have been taken from the corresponding references. Figure 2: The spin dynamical structure factor S ( q , ω ) calculated using DQMC for the Hubbard model. ( a ) False colour plots of the spectra along high symmetry directions in the Brillouin zone for different electron concentrations n . The calculations are done with the same Hubbard model parameters as in Fig. 1 . ( b ) Dispersion relations of the spin response peak in S ( q , ω) along these high symmetry directions for different n . ( c ) Comparison of the calculated and observed energies of the spectral peaks at selected momenta as a function of n ( t =400 meV has been used for the comparison). YBa 2 Cu 3 O 6+ x , YBa 2 Cu 4 O 8 and Nd 1.2 Ba 1.8 Cu 3 O 6+ x RIXS experimental data are taken from ref. 3 ; La 2− x Sr x CuO 4 RIXS experimental data are taken from ref. 6 . Error bars on the experimental data have been taken from the corresponding references. 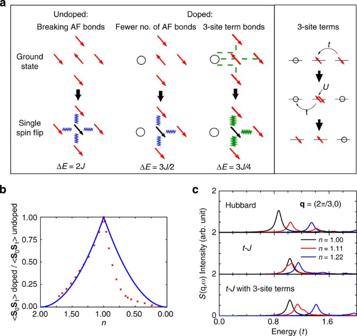Figure 3 Understanding doping dependence of the spin dynamical structure factorS(q, ω). (a) A cartoon illustrating the energy cost of spin excitations with doping within a ‘locally static hole’ model: (top row) ground state with AF correlations; (bottom row) a single spin-flip excitation. Green dashed lines represent the paths of hole delocalization by three-site terms, blue saw-tooth lines represent broken AF bonds and green saw-tooth lines represent broken three-site bonds. Undoped, a single spin-flip costs an energy of 2Jfrom the four broken AF bonds. With doping, this is reduced by the dilution of the AF background. With the three-site terms the overall energy cost increases compared with the undoped system due to the reduction in hole-delocalization energy. The side panel shows the process of hole-motion represented by the three-site terms, similar to the superexchange process. For electron doping, a particle-hole transformation can be applied so that a site with an open circle represents double occupancy. (b) Nearest neighbour spin-spin correlations 〈S0S1› as a function of electron concentrationnfrom DQMC. The solid lines represent a fit of the doping dependence in the ‘locally static hole’ model (see Methods). (c) A comparison between ED results forS(q, ω) inHHubbard,Ht−J, andHt−J+H3s(see Methods) for different values ofnat (2π/3, 0). The three-site terms lead to hardening of spin excitations in qualitative agreement with the results from the Hubbard model. We calculateS(q, ω) on the three model Hamiltonians with the parametersJ=0.4t,t=0.25t,U=10t(corresponding toJ=0.4tby the relationJ=4t2/U) and a Lorentzian broadening HWHM=0.05t. Full size image Figure 3 Understanding doping dependence of the spin dynamical structure factor S (q, ω) . ( a ) A cartoon illustrating the energy cost of spin excitations with doping within a ‘locally static hole’ model: (top row) ground state with AF correlations; (bottom row) a single spin-flip excitation. Green dashed lines represent the paths of hole delocalization by three-site terms, blue saw-tooth lines represent broken AF bonds and green saw-tooth lines represent broken three-site bonds. Undoped, a single spin-flip costs an energy of 2 J from the four broken AF bonds. With doping, this is reduced by the dilution of the AF background. With the three-site terms the overall energy cost increases compared with the undoped system due to the reduction in hole-delocalization energy. The side panel shows the process of hole-motion represented by the three-site terms, similar to the superexchange process. For electron doping, a particle-hole transformation can be applied so that a site with an open circle represents double occupancy. ( b ) Nearest neighbour spin-spin correlations 〈 S 0 S 1 › as a function of electron concentration n from DQMC. The solid lines represent a fit of the doping dependence in the ‘locally static hole’ model (see Methods). ( c ) A comparison between ED results for S ( q , ω) in H Hubbard , H t−J , and H t−J + H 3 s (see Methods) for different values of n at (2π/3, 0). The three-site terms lead to hardening of spin excitations in qualitative agreement with the results from the Hubbard model. We calculate S ( q , ω) on the three model Hamiltonians with the parameters J =0.4 t , t =0.25 t , U =10 t (corresponding to J =0.4 t by the relation J =4 t 2 / U ) and a Lorentzian broadening HWHM=0.05 t . Full size image We can address these points by considering the role of three-site exchange [16] , which lowers the system energy when both doped carriers and AF correlations are present (see Fig. 3a ). A local spin flip in an otherwise AF background produces a ferromagnetic alignment of nearest neighbour spins, which costs additional energy (of the same order as the spin exchange J =4 t 2 / U ) by suppressing hole- (or double-occupancy-) delocalization represented by the three-site terms. In fact, if we consider only the spin exchange contributions, the combined energy of a single-spin flip in the doped system (breaking both spin exchange and three-site bonds) is larger than that of the undoped system by ~ J /4 (see Fig. 3a ). This hardening has been observed in ED calculations of S ( q , ω) for the H Hubbard and H t−J + H 3 s Hamiltonians (see Methods) as shown in Fig. 3c upon electron doping. The situation is more subtle with hole doping, because this ‘locally static model’ no longer completely applies as seen in Fig. 3b . The negative next-nearest neighbour hopping t ′ (positive for electron doping) promotes magnetic sublattice mixing and a much larger destruction of the AF correlations [17] . With hole doping the trend observed in RIXS is fully recovered only in the Hubbard model, as shown in Fig. 2 , implying that higher order processes absent in t − J -type models become crucial in quantitatively reproducing the spin wave dispersion [18] . How do these results reconcile the seemingly contradictory observations between RIXS, neutron and Raman scattering? First, inelastic neutron scattering probes spin excitations particularly well around (π, π) momentum transfer, showing a vanishing spectral weight in the regime of large hole doping p ≃ 0.3 (refs 7 , 19 ). This behaviour is also visible in the numerical results presented in Fig. 2a , which suggest that the impact of doping on the intensity and dispersion of excitations near (0, 0) and (π, π) is not symmetric. The decreasing correlation length with doping, evidenced by the spin gap at (π, π) and the weak dispersion towards (π/2, π/2), thus impacts these momentum points more strongly than the AFZB paramagnons, in accordance with a locally static picture. Second, Raman scattering [8] , [20] , [21] shows a softening of the so-called bimagnon (double spin-flip or two-magnon) response upon both hole and electron doping. This trend has been reproduced by our ED calculations of the B 1 g Raman response shown in Fig. 4 (see Methods for the calculation details and the verification of bimagnon peaks). Strong magnon-magnon interactions reduce the bimagnon Raman peak energy from twice that of the single-magnon bandwidth as determined by AFZB magnons and quickly reduce the overall intensity. Taken as a whole, our results provide a qualitative, and in some cases quantitative, agreement with the salient experimental features of neutron scattering, Raman and RIXS measurements, suggesting that coherent propagating spin waves quickly disappear with the destruction of long-range AF order upon doping, while short-range, single spin-flip processes can survive to high doping levels as reflected in the evolution of S ( q , ω). Full polarization control will allow RIXS to become an effective tool for directly observing spin dynamics along the AFZB, particularly noting the electron/hole doping differences. Together with the dome-shaped superconducting phase diagram, these results imply that AFZB spin fluctuations might play a relatively minor role in the pairing mechanism, consistent with established experimental and numerical observations [22] , [23] , [24] . This calls into question a simple view of pairing that emphasizes only the spin exchange energy scale J . However, we suggest that a definitive resolution to this issue would come from future RIXS experiments along the BZ diagonal (out to (π/2, π/2)) to illuminate the evolution from antiferro- to ferro-magnetic correlations, compare with neutron scattering results and ultimately shed additional light on the intriguing mystery of cuprate high-temperature superconductivity. Numerical techniques We use exact diagonalization (ED) to evaluate the RIXS cross-section from the Kramers–Heisenberg formula [11] , spin dynamical structure factor S ( q , ω) and Raman scattering cross-section [25] on small clusters with periodic boundary conditions. We employ a 12-site Betts cluster [26] in evaluating the RIXS cross-section and S ( q , ω) shown in Fig. 1 . The Raman scattering response shown in Fig. 4 has been evaluated on 16- and 18-site square (or diamond-shaped) clusters, and the 18-site cluster was employed to evaluate S ( q , ω) for H Hubbard , H t−J and H t−J + H 3 s shown in Fig. 3 . The ED calculations for H Hubbard are performed with the Parallel ARnoldi PACKage (PARPACK) and the cross-sections obtained by use of the biconjugate gradient stabilized method and continued fraction expansion [12] . The ED calculations on H t−J and H t−J + H 3 s models are performed using the Lanczos algorithm. Finite temperature DQMC simulations [27] , [28] were performed on H Hubbard to obtain the imaginary time spin-spin correlation function from which the real frequency response function S ( q , ω) was obtained by analytic continuation using the maximum entropy method (MEM) [29] , [30] . These simulations were performed on 8 × 8 square lattice clusters with periodic boundary conditions at an inverse temperature β =3/ t for the same Hubbard Hamiltonian parameter values utilized in the ED studies. For this set of parameters, the DQMC method exhibits a significant fermion sign problem [31] over the entire doping range, which we address in the MEM [30] (see Supplementary Methods and Supplementary Fig. 6 ). MEM requires the use of a model function for determining an entropic prior in the analytic continuation routine. We utilize a Lorentzian model whose peak as a function of q is determined from a simple spin wave dispersion at small q out to the AFZB; however, beyond the AFZB the model assumes no softening as expected for long-range antiferromagnetism with the top of the magnon band set by approximations for the spin exchange J and an assumed reduction of the spin moment by quantum fluctuations. While some quantitative changes occur with significant changes to these default models, we have checked that the qualitative behaviour remains robust. The MEM routine returns the real frequency spin susceptibility from which S ( q , ω) is obtained from the fluctuation-dissipation theorem. More details about the models and numerical algorithms can be found in the following Methods and Supplementary Methods . 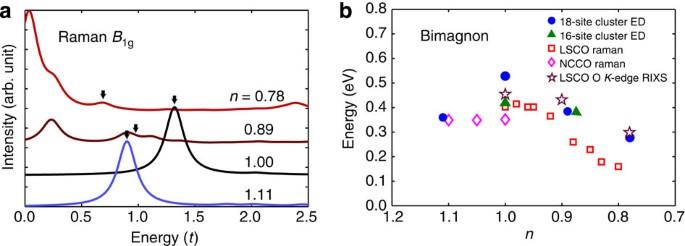Figure 4: Raman spectra as a function ofn. (a) TheB1gRaman spectra for various values ofncalculated using exact diagonalization of the Hubbard model on 18-site clusters (see Methods). The calculations are done with the same Hubbard model parameters as inFigs 1and2, and with a Lorentzian broadening HWHM=0.1t. Evolution of the spectral (‘bimagnon’) peak in the Raman spectra denoted by the black arrows (see Methods for identification of the ‘bimagnon’ peaks) in panel (a) together with the results from 16-site clusters (solid symbols). For the 18-site calculations, for example, the bimagnon peaks are obtained by fitting the spectra around the black arrow in panel (a) with Lorentzian functions. These results are compared with experiments (open symbols) obtained from Raman scattering on La2−xSrxCuO4(ref.20) and Nd2−xCexCuO4(ref.21), and oxygenK-edge RIXS on La2−xSrxCuO4(ref.36). Figure 4: Raman spectra as a function of n . ( a ) The B 1 g Raman spectra for various values of n calculated using exact diagonalization of the Hubbard model on 18-site clusters (see Methods). The calculations are done with the same Hubbard model parameters as in Figs 1 and 2 , and with a Lorentzian broadening HWHM=0.1 t . Evolution of the spectral (‘bimagnon’) peak in the Raman spectra denoted by the black arrows (see Methods for identification of the ‘bimagnon’ peaks) in panel ( a ) together with the results from 16-site clusters (solid symbols). For the 18-site calculations, for example, the bimagnon peaks are obtained by fitting the spectra around the black arrow in panel ( a ) with Lorentzian functions. These results are compared with experiments (open symbols) obtained from Raman scattering on La 2− x Sr x CuO 4 (ref. 20 ) and Nd 2− x Ce x CuO 4 (ref. 21 ), and oxygen K -edge RIXS on La 2− x Sr x CuO 4 (ref. 36 ). Full size image RIXS The Cu L 3 -edge RIXS cross-section is calculated using the Kramers–Heisenberg formula [11] for the single-band Hubbard model in which where q is the momentum transfer; ω in and ω= ω in − ω out are the incident photon energy (in our study the Cu L 3 -edge) and photon energy transfer, respectively; E 0 is the ground state energy of the system in the absence of a core-hole; |0› is the ground state wave function; (and h.c.) dictates the dipole transition process from Cu 2 p to the 3 d level (or from Cu 3 d to 2 p ), with the X-ray polarization either π or σ (the polarization vector parallel or perpendicular to the scattering plane); and Γ is the inverse core-hole lifetime (see Supplementary Note 2 ). In H Hubbard , <…> and … represent a sum over the nearest and next-nearest neighbour sites, respectively. The Hamiltonian for the intermediate state also involves the on-site energy for creating a 2 p core hole, Coulomb interaction U c induced by the core-hole and spin-orbit coupling λ , all denoted as in H CH . represents the spin-orbital coupling coefficients. The angle between the incident and the scattered photon propagation vectors is set to be 50°. The parameters used in the RIXS calculation are t =0.4 eV, U =8 t =3.2 eV, t ′=−0.3 t =−0.12 eV, , U c =−4 t =−1.6 eV, λ =13 eV and Γ =1 t =0.4 eV (refs 32 , 33 ). RIXS spectra at half-filling are taken only at the Cu L 3 resonance, and upon doping at the resonance closest to the half-filling Cu L 3 -edge resonant energy. The RIXS results were obtained for a Lorentzian broadening with half width at half maximum (HWHM)=0.01 eV (0.025 t ) and a Gaussian broadening with HWHM=0.047 eV (0.118 t ) on the energy transfer. The spin dynamical structure factor S ( q , ω), discussed in the next section, for H Hubbard was calculated using the same parameters to make comparison to our RIXS results. Spin dynamical structure factor The spin dynamical structure factor is defined as where we have studied the H Hubbard , H t−J and H t−J + H 3 s Hamiltonians: E 0 is the corresponding ground state energy of the model Hamiltonian; for H Hubbard ; , for H t−J and H 3 s ; ; and is restricted in the subspace without double occupancy and , in which the operator annihilates a dressed electron whose hopping conserves the number of effective doubly occupied sites [34] . To explore the similarities and differences between H Hubbard and H t−J (with and without H 3 s ), we calculate S ( q , ω) on the three model Hamiltonians with the parameters J =0.4 t , t ′=−0.25 t and U =10 t (corresponding to J =0.4 t by the relation J =4 t 2 / U ). Locally static model In the ‘locally static model’ (see Fig. 3b ) it is assumed that the holes destroy the short-range spin-spin correlations solely by the effect of ‘static’ doping, that is, by removing the spins and thus cutting spin bonds. In this case, the nearest neighbour spin-spin correlation can be calculated in the following way: where 〈 S 0 S 1 › is the abbreviation of 〈0| S i S j |0› for two neighbouring sites i and j , and p is the concentration of either doped holes ( P =1− n ) or doped electrons ( P = n −1). Raman scattering We calculate the Raman scattering cross-section in the B 1 g channel using the non-resonant response function for H Hubbard [25] : in which ? ( k )=−2 t ( cosk x + cosk y )−4 t ′ cosk x cosk y is the bare band dispersion, with parameters U =8 t and t ′=−0.3 t . t is taken as 0.4 eV to make comparison with experimental data. This two-particle response also has been studied recently in cluster dynamical mean-field theory [35] showing that, if calculated fully gauge invariantly, the nonresonant Raman B 1 g response shows the presence of a strong bimagnon peak at half filling. Nevertheless, the Raman spectrum calculated using this method for doped systems is sensitive to both charge and spin excitations in the low-energy regime. Our identification of the bimagnon excitations in the Raman spectra relies primarily on the qualitative evolution of the peaks in agreement with experimental observations [20] . We note that all of the excitations visible in our Raman spectra correspond to Δ S =0 transitions that have B 1 g symmetry. At half-filling, the energy of the excitation to which we assign bimagnon character lies within the charge gap, which makes the bimagnon assignment clear. Upon either hole or electron doping, we expect to develop charge excitations in the Raman response at low energy and for the two-magnon response to soften and decrease in intensity. Our assignment corresponds to an upper bound for the bimagnon energy scale with doping where the additional structure at low energies signals either charge excitations or a substantial broadening of the bimagnon excitations now represented by multiple features in the ED result (as discussed in connection with comparisons between DQMC and ED results). However, the energy scale clearly softens and, more importantly, the intensity drops (significantly) in agreement with the experimental observations where the bimagnon ‘peak’ becomes nearly impossible to distinguish from the charge background almost immediately upon crossing the AFM phase boundary. How to cite this article: Jia, C. J. et al. Persistent spin excitations in doped antiferromagnets revealed by resonant inelastic light scattering. Nat. Commun. 5:3314 doi: 10.1038/ncomms4314 (2014).